Direct and indirect Z-scheme heterostructure-coupled photosystem enabling cooperation of CO2reduction and H2O oxidation The stoichiometric photocatalytic reaction of CO 2 with H 2 O is one of the great challenges in photocatalysis. Here, we construct a Cu 2 O-Pt/SiC/IrO x composite by a controlled photodeposition and then an artificial photosynthetic system with Nafion membrane as diaphragm separating reduction and oxidation half-reactions. The artificial system exhibits excellent photocatalytic performance for CO 2 reduction to HCOOH and H 2 O oxidation to O 2 under visible light irradiation. The yields of HCOOH and O 2 meet almost stoichiometric ratio and are as high as 896.7 and 440.7 μmol g −1 h −1 , respectively. The high efficiencies of CO 2 reduction and H 2 O oxidation in the artificial system are attributed to both the direct Z-scheme electronic structure of Cu 2 O-Pt/SiC/IrO x and the indirect Z-scheme spatially separated reduction and oxidation units, which greatly prolong lifetime of photogenerated electrons and holes and prevent the backward reaction of products. This work provides an effective and feasible strategy to increase the efficiency of artificial photosynthesis. Solar-driven photocatalytic conversion of carbon dioxide (CO 2 ) to valuable organics or solar fuel is an attractive solution to both current energy and environment problems [1] , [2] , [3] , [4] . Reduction of CO 2 under visible light accounting for 45% sunlight energy by water rather than organic compound as an electron donor is the ultimate goal of photocatalysis. Enormous efforts have been devoted to developing a highly efficient photocatalyst for this prospect [5] , [6] , [7] . However, so far none of photocatalyst systems is satisfactory. Development of novel photocatalyst or system to realize highly efficient conversion of CO 2 remains the focus of future research. In various reduction products of CO 2 , including CO, HCOOH, CH 3 OH, HCHO, CH 4 , etc., HCOOH is a chemical with wide applications [8] , and even is considered as a promising bio-renewable feedstock for fine chemicals [9] . Although HCOOH as a two-electron-transfer product has the lowest degree of reduction among conversion products of CO 2 , all the reported photocatalysts to date still suffer from very low efficiency for HCOOH similar to other organic products [10] , [11] , [12] , [13] . This implies that the photocatalytic reduction of CO 2 to HCOOH is not easier than the reduction to other products. It is well known that the photocatalytic conversion of CO 2 with H 2 O involves two half-reactions, i.e. the reduction of CO 2 by the photogenerated electrons and protons, and the oxidation of H 2 O by the photogenerated holes. However, most of the reported photocatalysts could not catalyse simultaneously reduction of CO 2 to HCOOH and oxidation of H 2 O to O 2 [14] , and only work in the presence of organic hole-scavengers (e.g. triethanolamine (TEOA), trimethylamine (TEA), or ethylenediaminetetraacetic acid (EDTA)) [15] , [16] . Such photocatalytic CO 2 reduction at the cost of sacrificial electron donors is not sustainable and likely economically unsound. Even using hole scavenger, the photocatalysts only exhibit a formation rate of HCOOH with tens of micromoles, typically such as some metal-organic framework (MOF) materials (NH 2 -MIL-125(Ti), MIL-101(Fe)) [17] , [18] , inorganic–organic hybrid materials (a binuclear ruthenium(II) complex coupled with Ag/C 3 N 4 (ref. [19] , [20] ), Cu(I) complex photosensitized Mn(I) complex catalysts [21] ), and metal sulfide semiconductors ((Mo−Bi)S x /CdS) [22] . The C and Fe co-doped LaCoO 3 was reported to display an HCOOH yield up to 128 μmol g −1 h −1 without sacrificial reagent, but the oxidation product O 2 was not analysed [23] . Such photocatalytic CO 2 reduction without accompanying oxidation half-reaction is inexplicable. The photosynthesis essentially requires the stoichiometric photocatalytic CO 2 reduction and H 2 O oxidation which remains a great challenge in photocatalysis [24] . Silicon carbide (SiC), a metal-free semiconductor material, possesses a moderate wide band gap (2.4 eV) with an enough negative CB (ca. −1.1 V) to satisfy multielectron reactions of CO 2 reduction with H 2 O into carbon fuel and oxygen by solar energy [25] , [26] . So it has been considered as a promising photocatalyst for CO 2 conversion since the early research work [27] . However, the expected photocatalytic efficiency has not been achieved so far. This is due to very large difference between electron and hole migration rates in SiC (electron mobility 700 cm 2 V −1 s −1 , hole mobility 90 cm 2 V −1 s −1 ), which leads to the accumulation of photogenerated holes in the bulk and in turn suppresses the further generation of electrons under light irradiation. This makes the photogenerated carriers to be short-lived, especially the oxidation ability to be poor [28] , [29] . Moreover, the pristine SiC is lack of active sites for CO 2 adsorption and activation. Therefore, it is desirable to find the suitable cocatalysts to modify SiC. Additionally, the thermodynamically favourable backward reaction of the produced organics with oxygen on the photocatalyst surface is detrimental to decrease efficiency of CO 2 with pure H 2 O in the conversional one-pot reaction. These problems can be concurrently solved by constructing the multi-photocatalyst integration systems in which the oxidation and reduction reactions are independent in space but coupled in the transfer of photogenerated charges. Here, we report a Cu 2 O–Pt/SiC/IrO x hybrid photocatalyst, which is prepared by loading the photo-oxidation unit (IrO x ) and the photoreduction unit (Cu 2 O–Pt) on SiC surface. This configuration can enhance the lifetime of photogenerated charges and the CO 2 adsorption, and thus the photocatalytic efficiency. Furthermore, we construct a spatially separated reaction system consisting of two reaction chambers analogous to the natural photosynthetic systems. One chamber is loaded with the Cu 2 O–Pt/SiC/IrO x photocatalyst and Fe 2+ for CO 2 reduction, while the other chamber with the known Pt/WO 3 and Fe 3+ for H 2 O oxidation, and the two chambers are divided by a Nafion membrane that allows Fe 2+ and Fe 3+ ions to permeate through. This design facilitates H 2 O oxidation half-reaction and suppresses the backward reaction of the products. For the photocatalytic reaction of CO 2 with H 2 O to HCOOH and O 2 , the system shows very high photocatalytic efficiency under visible light irradiation. The HCOOH yield is as high as 896.7 μmol g −1 h −1 for the long-term reaction, 527 times higher than that of the pristine SiC (1.7 μmol g −1 h −1 ) in the conversional one-pot reaction. Most importantly, O 2 with a stoichiometric ratio is evolved concurrently. To the best of our knowledge, such high activity for reaction of CO 2 with pure H 2 O to HCOOH and O 2 is rarely reported before. 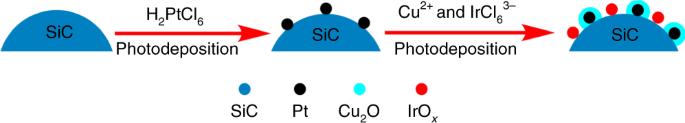Fig. 1: Formation process of Cu2O–Pt/SiC/IrOxby photodeposition. Schematic representation of Cu2O–Pt/SiC/IrOxsynthesis via controlled photodeposition. Configuration and composition of photocatalysts Figure 1 illustrates the formation process of the photocatalyst Cu 2 O–Pt/SiC/IrO x through the step-by-step photodeposition of Pt, Cu 2 O and IrO x on 3C-SiC (face centre cubic phase of SiC) surface. First, Pt nanoparticles were loaded onto SiC by a simple photodeposition to obtain Pt/SiC sample. Then the resulting Pt/SiC samples were dispersed in aqueous solution containing both Cu 2+ and IrCl 6 3− ions with UV light illumination, which led Cu 2+ to reduction into Cu 2 O species and IrCl 6 3− to oxidation into IrO x . Due to higher work function (5.6 eV) of Pt, the photogenerated electrons on SiC migrated to Pt and the photogenerated holes remained on SiC [30] , [31] . Thus the reduction reaction occurred on the Pt particle, while the oxidation reaction did on SiC. We thus concluded that the Cu 2 O was deposited on the Pt, while the IrO x on SiC. The resulting Cu 2 O–Pt and IrO x were located at different region of SiC surface. For comparison, the two reference samples, Cu 2 O–Pt/SiC and Pt/SiC/IrO x , were prepared also in the similar conditions with Cu 2+ -contained solution and IrCl 6 3− -contained solution, respectively. The loading amounts of cocatalysts on SiC samples were controlled by the photodeposition time (0.5–15 h) and then were quantified by a quadrupole inductively coupled plasma mass spectrometry (ICP-MS), as summarized in Supplementary Table 1 and Supplementary Note 1 . The contents of Pt, Cu 2 O and IrO x on the samples were controlled in the range of 0.83–2.6, 0.52–2.7 and 0.87–3.2 wt%, respectively. Based on the photocatalytic CO 2 reduction results, the optimal amount of Pt, Cu 2 O and IrO x is ascertained to be 1.3%, 1.8% and 2.2 wt% for Cu 2 O–Pt/SiC/IrO x photocatalyst, respectively. For the sake of brevity, hereafter the optimal photocatalyst with 1.3 wt% Pt, 1.8 wt% Cu 2 O and 2.2 wt% IrO x is referred simply to Cu 2 O–Pt/SiC/IrO x , unless specifically noted otherwise. Fig. 1: Formation process of Cu 2 O–Pt/SiC/IrO x by photodeposition. Schematic representation of Cu 2 O–Pt/SiC/IrO x synthesis via controlled photodeposition. Full size image The samples were firstly characterized by X-ray powder diffraction (XRD) (Supplementary Fig. 1 , Supplementary Note 2 ). For all samples, except the highly crystalline cubic phase SiC (JCPDS No. 65-0360), no XRD peaks corresponding to the cocatalysts (Pt, Cu 2 O and IrO x ) are observed due to their low contents and high dispersion on SiC surface. The BET specific surface area of SiC has a slight reduction from ~18 m 2 g −1 for bare SiC to ~14 m 2 g −1 for Cu 2 O–Pt/SiC/IrO x (Supplementary Fig. 2 , Supplementary Note 3 ), possibly because the cocatalysts with small-size particles block the micropore structure of SiC. The spatial locations of Pt, Cu 2 O and IrO x species on SiC surface were visualized by transmission electron microscopy (TEM) and HRTEM images (Fig. 2 ). The Pt nanoparticles have a uniform size of ca 2–4 nm and evenly distribute on the surface for all samples, as marked with yellow dotted circle (Fig. 2a , Supplementary Fig. 3 ). Cu 2 O was deposited over Pt nanoparticles to form a Cu 2 O–Pt intimate contact configuration for both Cu 2 O–Pt/SiC (Supplementary Fig. 3c , Supplementary Note 4 ) and Cu 2 O–Pt/SiC/IrO x samples (Fig. 2a ) as marked with red circle, while the IrO x species are not deposited at the same location as Cu 2 O–Pt species for both Pt/SiC/IrO x (Supplementary Fig. 3d ) and Cu 2 O–Pt/SiC/IrO x samples (Fig. 2a ), as marked with blue dotted circle. The lattice spacings of Cu 2 O–Pt/SiC/IrO x samples (Fig. 2b , Supplementary Fig. 3 ) are 0.252, 0.226, 0.211 and 0.260 nm assigning to the (111) facet of SiC, (111) facet of Pt, (200) facet of Cu 2 O and (101) facet of IrO 2 (refs. [32] , [33] , [34] , [35] ), respectively. The Cu 2 O–Pt intimate contact structure is further testified by STEM-EDS mapping (Fig. 2c , Supplementary Fig. 4 ). In the selected area, Pt has the same distribution and appears at almost the same position as Cu, further demonstrating the deposition of Cu 2 O over Pt particles. Nevertheless, there is also a part of Cu to be deposited on SiC surface. IrO x looks like a random deposition on the entire surface of SiC due to very small cluster particles, but it is separated from Cu 2 O–Pt on the SiC surface, because the distribution of Ir-L in mapping images (Supplementary Fig. 5 , Supplementary Note 4 , Fig. 2c ) has an obvious difference from that of other elements through careful comparison. Fig. 2: Spatial location of cocatalysts. a TEM, b HRTEM images and c STEM image and corresponding EDS mapping profiles for C-K, Si-K, Pt-L, Cu-K and Ir-L of Cu 2 O–Pt/SiC/IrO x . Full size image The chemical composition distribution of the outermost layer on SiC surface was further analysed by a high-sensitivity low-energy ion scattering (HS-LEIS) studies. 3 keV 4 He + HS-LEIS spectra (Fig. 3a ) give the signal of the light elements on the outer surface (such as C, O and Si), but have poor sensitivity to Cu, Pt and Ir heavy elements. Figure 3b shows the 5 keV 20 Ne + HS-LEIS spectra of SiC, Pt/SiC, Cu 2 O–Pt/SiC, Pt/SiC/IrO x and Cu 2 O–Pt/SiC/IrO x . 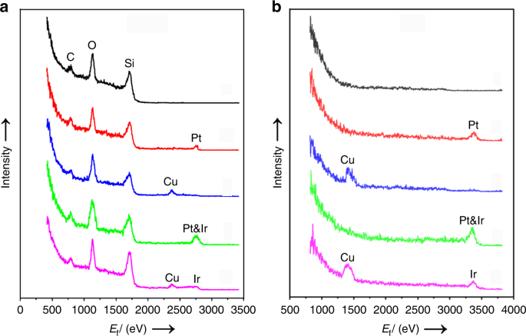Fig. 3: The chemical composition on the outermost surface. HS-LEIS spectra usinga3 keV4He+andb5 keV20Ne+for the samples: SiC (black), Pt/SiC (red), Cu2O–Pt/SiC (blue), Pt/SiC/IrOx(green) and Cu2O–Pt/SiC/IrOx(pink). Pt element is detected on the outmost surface for Pt/SiC. Only Cu element is observed on Cu 2 O–Pt/SiC, clearly indicating that Cu 2 O is deposited on the surface of Pt nanoparticles. Although HS-LEIS peaks of Pt and Ir cannot be resolved using 5 keV 20 Ne + because their atomic mass is too close, it should be noted that intensity of the fused peaks of Pt and Ir at 3367 eV for Pt/SiC/IrO x is significantly stronger than that of sole Pt peak in Pt/SiC. This indicates that both IrO x and Pt coexist on the outermost surface of Pt/SiC/IrO x . However, the peak at 3367 eV for Cu 2 O–Pt/SiC/IrO x samples weakens significantly as compared with Pt/SiC/IrO x . Since Pt is covered by Cu 2 O in Cu 2 O–Pt/SiC/IrO x , the low peak at 3367 eV of Cu 2 O–Pt/SiC/IrO x can be only assigned to IrO x on the outermost surface. Therefore, the HS-LEIS results constitute another strong evidence that the Cu 2 O–Pt and IrO x cocatalysts are spatially separated on SiC surface for Cu 2 O–Pt/SiC/IrO x . Fig. 3: The chemical composition on the outermost surface. HS-LEIS spectra using a 3 keV 4 He + and b 5 keV 20 Ne + for the samples: SiC (black), Pt/SiC (red), Cu 2 O–Pt/SiC (blue), Pt/SiC/IrO x (green) and Cu 2 O–Pt/SiC/IrO x (pink). Full size image The chemical states of the Pt, Cu and Ir elements in samples were analysed by XPS (Fig. 4 ). 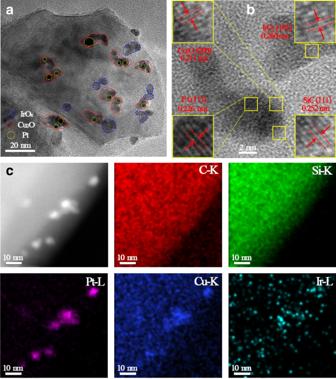Three sets of Pt 4 f XPS peaks can be assigned to metallic Pt 0 and partially oxidized Pt 2+ and Pt 4+ species [36] . Fig. 2: Spatial location of cocatalysts. aTEM,bHRTEM images andcSTEM image and corresponding EDS mapping profiles for C-K, Si-K, Pt-L, Cu-K and Ir-L of Cu2O–Pt/SiC/IrOx. The ratio of Pt 0 is calculated to be accounting for 70 ± 4% of the sum Pt species for the all Pt-contained samples (Supplementary Table 2 ). Cu species and Ir species are mainly in the state of Cu 2 O and mixed valence oxides (IrO x ), respectively [37] , [38] . Nevertheless, the binding energies (BE) of Pt, Cu or Ir have obvious differences among samples. For Pt/SiC, the BE of Pt 4 f 7/2 and Pt 4 f 5/2 are respectively 70.8 and 74.1 eV, which are lower than that of the pure metallic Pt (Pt 4 f 7/2 = 71.2 eV) [39] . This is because the electron transfer occurs from the SiC substrate to Pt particles with higher work function [40] , [41] . When Cu 2 O is subsequently deposited on Pt/SiC to form Cu 2 O–Pt/SiC, the BE of Pt 4 f 7/2 shifts towards higher energy (71.1 eV), but is still slight lower than that of metallic Pt, indicating the electron transfer still from SiC to Cu 2 O under mediation of Pt nanoparticles. On the contrary, when IrO x is deposited onto Pt/SiC to form Pt/SiC/IrO x , the BE of Pt 4 f shifts to lower position. This indicates that IrO x deposition induces the electron transfer from IrO x to the SiC surface and thus enhances the electron transfer to Pt particles. In the case of the co-deposition of IrO x and Cu 2 O on Pt/SiC, the BE of Pt 4 f in Cu 2 O–Pt/SiC/IrO x is comparable with Cu 2 O–Pt/SiC. This demonstrates that the electrons are finally transferred from both SiC and IrO x into Cu 2 O. As a result, the BE of Cu 2 p for Cu 2 O–Pt/SiC/IrO x is also lower than that of Cu 2 O–Pt/SiC. In reverse, the BE of Ir 4 f for Cu 2 O–Pt/SiC/IrO x is slightly positively shifted as compared with Pt/SiC/IrO x . The above results show the existence of the strong interfacial interaction between co-catalyst and SiC, which would be favourable for the electron migration and transfer in Cu 2 O–Pt/SiC/IrO x . Fig. 4: The chemical states of cocatalysts. a Pt 4 f XPS spectra, b Cu 2 p XPS spectra, and c Ir 4 f XPS spectra of Pt/SiC, Cu 2 O–Pt/SiC, Pt/SiC/IrO x and Cu 2 O–Pt/SiC/IrO x samples. Full size image Photocatalytic performance of CO 2 reduction with H 2 O The photocatalytic CO 2 reduction was performed in the spatially separated reaction system. Fe 2+ and Fe 3+ were added respectively in the CO 2 -reduction compartment and the H 2 O-oxidation compartment in the beginning of the reaction (see Supplementary Fig. 6 ) [42] , [43] . During the photoreaction process, Fe 3+ and Fe 2+ ions are able to permeate through the Nafion membrane driven by the concentration gradient. The photocatalytic activities of the samples for the reaction of CO 2 with H 2 O were tested under visible light irradiation in order to find out the optimal contents of cocatalysts, as shown in Fig. 5 and Supplementary Table 1 . HCOOH is detected as a main product for all photocatalysts. The bare SiC only shows 24.1 μmol g −1 h −1 of HCOOH yield. Over Pt/SiC samples, the HCOOH yield shows a volcanic curve with increasing Pt contents and the highest HCOOH yield (57.7 μmol g −1 h −1 ) occurs at 1.3 wt% Pt content (Fig. 5a ). On the Cu 2 O–Pt/SiC sample with 1.3 wt% Pt, the product HCOOH shows the highest yield (304.6 μmol g −1 h −1 ) at 1.8 wt% content of Cu 2 O (Fig. 5b ). On the Pt/SiC/IrO x with the optimum Pt content (1.3 wt%), the optimal loading content of IrO x is 2.2 wt% at which the HCOOH yield is ca. 472.0 μmol g −1 h −1 (Fig. 5c ). When both IrO x and Cu 2 O are simultaneously deposited on the optimal Pt/SiC, the highest yield of HCOOH, 896.7 μmol g −1 h −1 , occurs at ca. 2.2 wt% of IrO x and 1.8 wt% of Cu 2 O. When Cu 2 O content is higher than 1.8 wt%, further increasing Cu 2 O photodeposition induces more amount of Cu 2 O on both Pt particles and the exposed SiC surface. The deposited Cu 2 O on SiC could block the optical absorption of SiC, and an over-thick Cu 2 O layer on Pt surface is also unfavourable to CO 2 reduction on Cu 2 O–Pt [32] . The higher IrO x contents <2.2 wt%, the more active sites of IrO x are provided to enhance the Fe 2+ oxidation. However, an excess amount of IrO x may lead to the growth of IrO x into large particles on SiC surface, which is harmful to the photocatalytic reaction. The HCOOH yield over the optimal Cu 2 O–Pt/SiC/IrO x is almost 37 times of the activity of the bare SiC. To the best of our knowledge, the photocatalytic efficiency of our system is substantially higher than that of other various photocatalysts reported so far (seen activity comparison in Supplementary Table 3 ). Fig. 5: The optimal contents of cocatalysts for CO 2 reduction. Change in HCOOH evolution rate a on Pt/SiC with increasing Pt content, b on Cu 2 O–Pt (1.3 wt%)/SiC with increasing Cu 2 O, c on Pt (1.3 wt%)/SiC/IrO x with increasing IrO x , and d on Cu 2 O–Pt/SiC/IrO x with increasing Cu 2 O and IrO x , in spatially separated reactor under visible light irradiation. Reaction conditions: 50 mg SiC-based photocatalyst and 300 mL of 2 mM FeCl 2 aqueous solution were placed in the CO 2 -reduction chamber, 100 mg Pt/WO 3 and 300 mL of 2 mM FeCl 3 aqueous solution in the H 2 O oxidation chamber, the pH of solution was adjusted to 2.3 by adding hydrochloric acid to prevent precipitation of the iron ions aqueous solution. Full size image O 2 is confirmed as main product evolving in the Pt/WO 3 oxidation chamber of the separated reaction system. Figure 6a shows the production of O 2 in the Pt/WO 3 chamber and HCOOH in the Cu 2 O–Pt/SiC/IrO x chamber vs. irradiation time. Both yields of HCOOH and O 2 increase linearly, and reach 7200 and 3300 μmol g −1 during 8 h photocatalytic reactions, respectively. 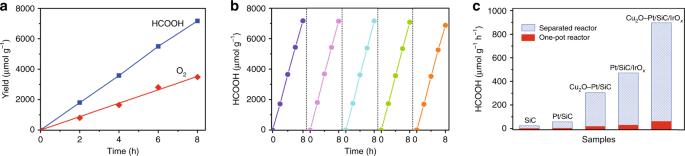Fig. 6: Photocatalytic performance of CO2reduction with H2O. aEvolutions of HCOOH and O2as a function of illumination time andbcycle experiment of HCOOH evolution in the spatially separated reaction system with Cu2O–Pt/SiC/IrOxas the reduction side photocatalyst.cComparison for the HCOOH evolution between in the spatially separated reaction system and in the conventional one-pot reactor with different samples as the reduction side photocatalyst. Moreover, the ratio of product O 2 to HCOOH is close to the stoichiometric number of reaction (2CO 2 + 2H 2 O → 2HCOOH + O 2 ) in the whole process. Influence of the Pt amount of Pt/WO 3 on the photocatalytic O 2 and HCOOH evolutions in the separated reaction system was also investigated (Supplementary Fig. 7 ). As decreasing Pt content to 0.5 wt% of Pt/WO 3 , the O 2 and HCOOH yields decrease to 296.6 and 618.7 μmol g −1 h −1 , respectively. However, the ratio of O 2 to HCOOH is still close to the stoichiometric number. When the Pt content increases to 1.5 wt%, both O 2 and HCOOH evolution is almost the same as that of 1.0 wt% Pt. The 1.0 wt% Pt content is optimal for the Pt/WO 3 in the separated reaction system. Obviously, Pt content of Pt/WO 3 does not affect the stoichiometric ratio of product HCOOH to O 2 . This is because Fe 3+ /Fe 2+ redox couple acts as the electron transfer medium between CO 2 reduction and H 2 O oxidation by the concentration diffusion through the Nafion membrane, which makes the reaction stoichiometrically proceeded in the reaction process. However, the HCOOH yield shows a downtrend as prolonging the reaction time (Supplementary Fig. 8 ). The decrease of activity is because pH value of the reaction solution is increased from 2.3 at the initial stage to 4.5 after 12 h reaction along with the consumption of H + in the process of CO 2 reduction. The increase in solution alkalinity can result in hydrolysis of Fe 3+ to FeOOH or Fe(OH) 3 , as confirmed by the Fe 2 p XPS spectrum of the sample after the reaction (Supplementary Fig. 9 ). However, the activity is highly stable in five cycles of total 40 h (Fig. 6b ) when the Cu 2 O–Pt/SiC/IrO x is centrifuged out and then added to the fresh solution before each new cycle. Therefore, the increase in solution alkalinity during the photocatalytic reaction is one of reasons effecting stability of the reaction, which should be avoided by increasing solution acidity. Fig. 6: Photocatalytic performance of CO 2 reduction with H 2 O. a Evolutions of HCOOH and O 2 as a function of illumination time and b cycle experiment of HCOOH evolution in the spatially separated reaction system with Cu 2 O–Pt/SiC/IrO x as the reduction side photocatalyst. c Comparison for the HCOOH evolution between in the spatially separated reaction system and in the conventional one-pot reactor with different samples as the reduction side photocatalyst. Full size image The Cu 2 O–Pt/SiC/IrO x samples before and after the photocatalytic reaction were characterized by XPS (Supplementary Fig. 10 ), indicating some differences in chemical states of Pt, Ir and Cu. However, the changes of metal states are likely to have no significantly influence or be not main factor on the photocatalytic activity stability. (i) For Pt, the XPS Pt 4 f peaks narrow down and the shoulder peaks become weak for the used sample, but the BE values of main peaks keep almost unchanged before and after the photocatalytic reaction. The main peaks at the BEs of 74.7 eV (Pt 4 f 5/2) and 71.5 eV (Pt 4 f 7/2) are attributed to Pt(0). The shoulder peaks are belonged to Pt 2+ and Pt 4+ species. It can be seen that a part of high valence Pt species were translated also into Pt (0) after longtime reaction, which could be beneficial to the photocatalysis. (ii) For IrO x , the Ir 4 f peaks not only become narrow but also shift towards lower energy after the photocatalytic reaction. The wide Ir 4 f peaks of both the fresh and the used samples cover Ir 0 , Ir 3+ and Ir 4+ species, indicating the mix valence state feature of IrO x . Accordingly, the Ir 4 f 7/2 peak can be deconvoluted into a contribution of Ir 0 (61.3 eV), Ir 4+ (62.4 eV) and Ir 3+ (63.5 eV) species [44] , [45] , [46] . 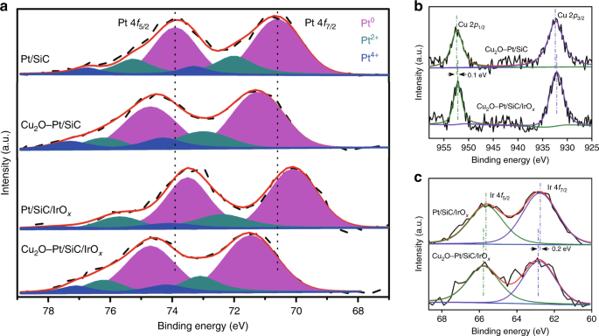The phenomena are universal for Ir-loaded catalysts, which is also the reason why iridium oxide is usually be expressed as IrO x rather than IrO 2 [47] . Fig. 4: The chemical states of cocatalysts. aPt 4fXPS spectra,bCu 2pXPS spectra, andcIr 4fXPS spectra of Pt/SiC, Cu2O–Pt/SiC, Pt/SiC/IrOxand Cu2O–Pt/SiC/IrOxsamples. It is estimated from the peak intensities that the contents of Ir 4+ are increased, while Ir 3+ contents are decreased in the used sample as compared with the fresh sample (see Supplementary Table 4 ). Such a change in the Ir 4 f XPS spectra can be explained by the changes in the crystallinity and coordination numbers [48] , [49] . For the fresh sample, the broader and higher BE peaks suggest the existence of partial amorphous or high oxygen coordinated Ir species. For the used sample, the shift of BE of Ir 4 f peak towards lower energy indicates an increase in the rutile phase IrO 2 during the photocatalytic process since the IrO x could be mainly excited from the d(t 2g ) to the d(e g ) band (1.5–2.75 eV) under visible light irradiation based on the literature [50] . It is possible that the change in Ir valence state or crystallinity do not affect the photoinduced d–d transition and thus photocatalytic performance. (iii) As for Cu 2 O, the Cu 2 p XPS spectrum shows a minor change. The BEs of the main peaks of Cu 2 p remain almost the same before and after the reaction, only a minuscule shift towards lower energy. We could not exclude the possibility that a small amount of Cu(I) was translated into Cu(0) after the photocatalytic reaction. Because some Cu 2 O is deposited synchronously on the SiC surface, the small change of Cu valence state can occur partly for these Cu 2 O species, which could have no remarkable influence on the photocatalytic performance. Other two control experiments were carried out also. When 13 CO 2 instead of CO 2 was used as a reactant, 13 C NMR analysis for the reaction solution verifies that only a strong peak at 171.5 ppm attributed to the 13 C in H 13 COOH was observed (Supplementary Fig. 11 ) [51] . When CO 2 was not added in the reaction system, no HCOOH was detected. These results show that the product HCOOH is formed from the photocatalytic CO 2 reduction. As H 2 18 O instead of H 2 O is used as the reactant in a small dose simulated reaction, the mass spectroscopy analysis gives a main peak at m / z = 36 corresponding to 18 O 2 (Supplementary Fig. 12 ), confirming the product O 2 originating from H 2 O oxidation. Careful analysis reveals that except HCOOH no carbon-containing products, such as CO, HCHO and CH 4 , come into being in the gas phase. Nevertheless, there is only a very slight amount of H 2 to evolve as a by-product (Supplementary Fig. 13 ), implying existence of competition between the reduction of H + to H 2 and the reduction of CO 2 to HCOOH by photogenerated electrons. In the absence of CO 2 atmosphere, however, only a slightly enhanced amount of H 2 evolves in the gas phase (Supplementary Fig. 14 ), although the photocatalytic reaction is performed in the acidic aqueous solution. This indicates that the SiC-based photocatalyst is not good for H 2 evolution from water, which may be because that it lacks the active sites or has high overpotential for the H 2 evolution. However, for the reduction of CO 2 , the SiC-based photocatalyst can be particularly effective. The photocatalytic activity for the reaction of CO 2 with H 2 O was also evaluated in the conventional one-pot reactor, where we added simultaneously SiC-based catalyst, Pt/WO 3 and Fe 2+ /Fe 3+ . 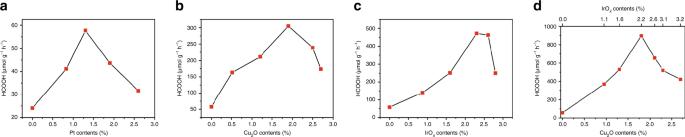HCOOH and O 2 are also detected as main products. Fig. 5: The optimal contents of cocatalysts for CO2reduction. Change in HCOOH evolution rateaon Pt/SiC with increasing Pt content,bon Cu2O–Pt (1.3 wt%)/SiC with increasing Cu2O,con Pt (1.3 wt%)/SiC/IrOxwith increasing IrOx, anddon Cu2O–Pt/SiC/IrOxwith increasing Cu2O and IrOx, in spatially separated reactor under visible light irradiation. Reaction conditions: 50 mg SiC-based photocatalyst and 300 mL of 2 mM FeCl2aqueous solution were placed in the CO2-reduction chamber, 100 mg Pt/WO3and 300 mL of 2 mM FeCl3aqueous solution in the H2O oxidation chamber, the pH of solution was adjusted to 2.3 by adding hydrochloric acid to prevent precipitation of the iron ions aqueous solution. Figure 6c compares the HCOOH yields under two different reaction modes (see also Supplementary Table 5 ). It can be seen that all the samples show much higher HCOOH yield with the spatially separated reaction system than with the one-pot reaction mode. For SiC, Pt/SiC, Cu 2 O–Pt/SiC, Pt/SiC/IrO x and Cu 2 O–Pt/SiC/IrO x photocatalyst, the HCOOH yield is 1.7, 3.5, 18.6, 30.4 and 61.5 μmol g −1 h −1 with the one-pot reaction, while it is 24.1, 57.7, 304.6, 472.0 and 896.6 μmol g −1 h −1 with the spatially separated system, respectively. Obviously, the photocatalytic activity of the spatially separated system is ca ~ 15 times higher than that in the one-pot reaction reactor for each photocatalyst. In the one-pot reaction system, the backward reaction of HCOOH re-oxidization by O 2 should be one of the reasons for the low evolution of HCOOH and O 2 . Both Fe 3+ competing with CO 2 for the generated electrons and Fe 2+ competing with H 2 O for the photogenerated holes could also take place at the same time. However, the effects of the later could be weaker than that of the former, because the evolutions of HCOOH and O 2 are lower if no adding Fe 3+ and Fe 2+ (see the first column in Supplementary Table 5 ). This could be one of reasons for high efficiency of the spatially separated system. However, the reasonableness of this inference requires the following two premises: the product HCOOH (i) does not diffuse to the oxygen evolution chamber from the reduction chamber through the Nafion membrane and (ii) is not oxidized in the reduction chamber by the Fe 3+ , with increase in the production of HCOOH. Accordingly, two additional experiments were done. The permeation of HCOOH across the Nafion membrane from the HCOOH solution (1200 μmol L −1 , corresponding to the maximum yield of HCOOH in the separated system for 8 h reaction) to pure H 2 O is determined firstly. Only very limited amount of HCOOH (<5%) is diffused to the pure water across the Nafion membrane within 8 h (Supplementary Fig. 15 ). Another experiment is the solution (pH = 2.3) with HCOOH (1200 μmol L −1 ) and Fe 2+ /Fe 3+ (2 mmol L −1 ) under visible light illumination. The concentration of HCOOH remains almost unchanged (Supplementary Fig. 16 ). These indicate that our new system is indeed effective to prevent the backward reaction. The wavelength-dependent evolution of HCOOH was also performed to gain the apparent quantum yield (AQY) (Supplementary Fig. 17 ). Obviously, the AQY of HCOOH evolution on the optimal Cu 2 O–Pt/SiC/IrO x sample is well matched with the optical absorption spectra. Under 400 nm light irradiation, the AQY of HCOOH evolution can be reached near 1.44%. The in situ CO 2 adsorption FT-IR spectra The photocatalytic activity of Cu 2 O–Pt/SiC/IrO x is always higher than that of the other samples both in the spatially separated system and in the one-pot reactor. The HCOOH yield on the optimal Cu 2 O–Pt/SiC/IrO x sample in the spatially separated system is 37 and 527 times higher than that on the bare SiC in the spatially separated system and in the one-pot reactor, respectively. Obviously, the high efficiency of Cu 2 O–Pt/SiC/IrO x for the reaction of CO 2 with H 2 O to HCOOH can be related to the photocatalyst surface feature. The in situ CO 2 adsorption FT-IR spectra were measured to gain insight into the effect of surface feature. As shown in Fig. 7a , all photocatalysts show the multiple IR adsorption peaks of CO 2 in the range of 2200–2500 cm −1 in the dark. It is noteworthy that both the samples containing Cu, i.e. Cu 2 O–Pt/SiC and Cu 2 O–Pt/SiC/IrO x , show much stronger CO 2 adsorption band than nude SiC, Pt/SiC and Pt/SiC/IrO x . This implies that CO 2 molecules are mainly adsorbed on the Cu 2 O co-catalyst in Cu 2 O–Pt/SiC and Cu 2 O–Pt/SiC/IrO x [32] , [52] . 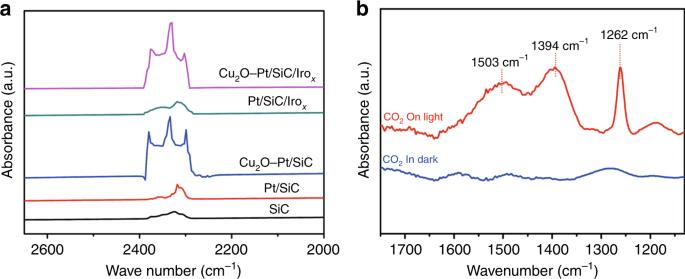Fig. 7: Adsorption of CO2on photocatalysts. aIn situ FT-IR spectra of CO2adsorbed on different photocatalysts.bIn situ FT-IR spectra of CO2adsorbed on Cu2O–Pt/SiC/IrOxbefore and after visible light irradiation. All the spectra are the difference spectra between after and before CO2adsorption. Figure 7b shows the in situ CO 2 adsorption FT-IR spectra on Cu 2 O–Pt/SiC/IrO x in the range of 1700–1200 cm −1 after and before light irradiation, which is a reflection of chemical adsorption. No absorption attributable to C–O species appears on Cu 2 O–Pt/SiC/IrO x in the absence of CO 2 gas (omitted). As introduction of CO 2 , Cu 2 O–Pt/SiC/IrO x shows very weak several absorption peaks before visible light irradiation. However, three strong absorption bands appear upon visible light irradiation. Both the wide absorption band at 1394 cm −1 and the weak band at 1503 cm −1 are ascribed to bidentate carbonate species bonded to the Cu 2 O surface, while the absorption band at 1262 cm −1 is assigned to a monodentate carbonate to the Cu 2 O surface [53] , [54] . This demonstrates that CO 2 molecules are activated at room temperature by the Cu 2 O co-catalyst on Cu 2 O–Pt/SiC/IrO x surface under light irradiation. Moreover, the acidic aqueous solution (pH = 2.3) is helpful for formation of the carboxyl radical intermediate (·COOH) or the formate anion (HCOO − ) that is further easily converted into HCOOH [14] , [55] . This could be the second possible reason for the high efficiency of the spatially separated system. High selectivity of product HCOOH may be related to the different reaction mechanism dependent on the reaction conditions, such as the photocatalyst states (defects, crystal faces, doping, etc. ), reaction conditions (temperature, pH, CO 2 concentration, reactant phase, etc. ), co-catalyst and so on. In the gas (CO 2 , H 2 O vapour)–solid (catalyst.) mode, it has been found that the SiC-based composite (MoS 2 /SiC) photocatalyzed the CO 2 reduction into CH 4 undergoing HCOOH, HCHO and CH 3 OH intermediates on SiC surface by the hydrogenation pathways [26] . In the present work, the reaction is conducted in gas (CO 2 )–liquid (H 2 O)–solid(catalyst) mode and the acidic aqueous solution. In addition, the reduction of CO 2 occurs on the Cu 2 O sites rather than SiC, which is helpful for formation of the carboxyl (hydroxyformyl) radical intermediate · COOH and HCOOH [14] , [56] . Fig. 7: Adsorption of CO 2 on photocatalysts. a In situ FT-IR spectra of CO 2 adsorbed on different photocatalysts. b In situ FT-IR spectra of CO 2 adsorbed on Cu 2 O–Pt/SiC/IrO x before and after visible light irradiation. All the spectra are the difference spectra between after and before CO 2 adsorption. Full size image Photoelectrochemical properties of Cu 2 O–Pt/SiC/IrO x The photoelectrochemical responses and the photoluminescence spectra of these photocatalysts were measured. 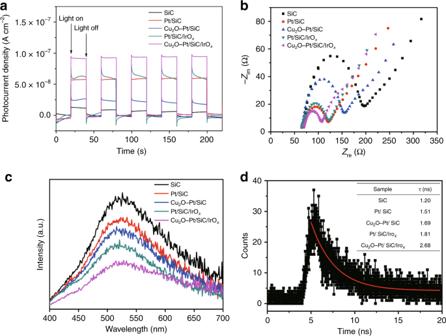Fig. 8: Separation efficiency and lifetime of carriers. aPeriodic on/off photocurrent response,bAC Impedance andcPL (photoluminescence) spectra for different photocatalysts.dTime-resolved photoluminescence spectroscopy of Cu2O–Pt/SiC/IrOx. 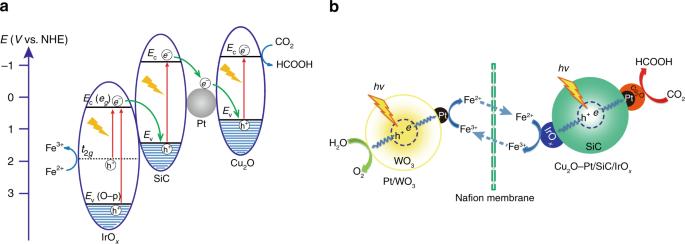Fig. 9: Electronic structure and photocatalytic mechanism. aThe electron transfer processes in Cu2O–Pt/SiC/IrOxunder light illumination.bThe proposed mechanism of the separated system for the efficient CO2reduction and O2evolution. Figure 8a, b shows the photocurrents and AC impedance of the different samples. The photocurrents increase in order of SiC, Cu 2 O–Pt/SiC, Pt/SiC, Pt/SiC/IrO x and Cu 2 O–Pt/SiC/IrO x , and the AC impedance values decrease in the same order. Obviously, Cu 2 O–Pt/SiC/IrO x shows the biggest photocurrent and the smallest AC impedance, indicating the highest electron transfer rate and separation efficiency. However, the sample Cu 2 O–Pt/SiC and Pt/SiC show a slight abnormality, i.e. both the photocurrent increase order and the AC impedance decrease order are inconsistent with the increase order of photocatalytic activity. This can be explained by the dependence of photocatalytic activity on not only the transfer rate and separation efficiency of photogenerated charges but also the surface chemistry characteristics of photocatalyst. Figure 8c is the steady-state photoluminescence (PL) spectra of these samples. The PL intensities decrease in accordance with the order of SiC, Pt/SiC, Cu 2 O–Pt/SiC, Pt/SiC/IrO x and Cu 2 O–Pt/SiC/IrO x , which agree with the change in the photocatalytic activity. Since low PL intensity corresponds to low recombination rate of photogenerated charges, the lowest PL intensity indicates the smallest recombination rate of photogenerated charge for Cu 2 O–Pt/SiC/IrO x . Figure 8d shows the time-resolved photoluminescence spectroscopy of these samples (see detailed Supplementary Fig. 18 ), and the corresponding average lifetimes ( τ ) of charge carriers (the inset table). The τ value of nude SiC is about 1.2 ns, consistent with the reported literature [57] . Loading Pt, Cu 2 O and IrO x nanoparticles lead to an increase in the lifetime τ . In these samples, Cu 2 O–Pt/SiC/IrO x has the highest τ value. The increase in the lifetime τ of the charge carriers could increase the probability of their involvement in photocatalytic reactions before recombination [58] , [59] , [60] . So, increases in the transfer rate, separation efficiency and lifetime of photogenerated charges could be the third reason for high efficiency of the spatially separated system. Fig. 8: Separation efficiency and lifetime of carriers. a Periodic on/off photocurrent response, b AC Impedance and c PL (photoluminescence) spectra for different photocatalysts. d Time-resolved photoluminescence spectroscopy of Cu 2 O–Pt/SiC/IrO x . Full size image Photocatalytic mechanism of the spatially separated system The next issue is the electron structure of Cu 2 O–Pt/SiC/IrO x and the photocatalytic mechanism of the spatially separated system. The electron structure parameters of SiC and Cu 2 O were reckoned by combination of the UV–Vis diffuse reflection spectra with the Mott-Schottky analysis (Supplementary Fig. 19 ). The optical absorption edge of the nude SiC is at 501 nm. The band gap energy and the conduction band (CB) potential of SiC are ca. 2.48 eV and −1.08 V (vs. SHE), respectively. The parent Cu 2 O is estimated to have a band gap of 1.98 eV and CB of −1.28 V. It has been reported that the IrO x could be excited from the d(t 2g ) to the d(e g ) band (1.5–2.75 eV) by visible irradiation and from the O-p band to the d(e g ) (>3.0 eV) band by ultraviolet irradiation, and its CB is +0.35 V [50] . For the Cu 2 O–Pt/SiC/IrO x photocatalyst, Cu 2 O–Pt and IrO x cocatalysts are separated each other on SiC surface, and Pt is sandwiched between Cu 2 O and SiC. Thus, Cu 2 O–Pt/SiC/IrO x is suggested to have the energy band alignment in Fig. 9a . Fig. 9: Electronic structure and photocatalytic mechanism. a The electron transfer processes in Cu 2 O–Pt/SiC/IrO x under light illumination. b The proposed mechanism of the separated system for the efficient CO 2 reduction and O 2 evolution. Full size image If the Cu 2 O co-catalyst directly contacts with SiC without Pt, the photoelectron transfers on the resulting Cu 2 O/SiC composite is speculated to follow the Z-scheme transfer from SiC to Cu 2 O, which has been reported in many literatures [61] , [62] , [63] . Such Z-scheme photoelectron transfer was verified by a photocatalytic probe reaction. When the water solution containing the Cu 2 O/SiC sample and H 2 PtCl 6 was illuminated by UV light, the reduction reaction (PtCl 6 2− + 4 e − → Pt + 6Cl − ) would occur on the Cu 2 O/SiC surface. The TEM image clearly indicates preponderant photodeposition of Pt particles over Cu 2 O particle rather than over SiC surface (Supplementary Fig. 20 ), unambiguously verifying the Z-scheme electron transfer, i.e. the transfer of photogenerated electron from the CB of SiC to the VB of Cu 2 O. For our Cu 2 O–Pt/SiC/IrO x sample, we can reasonably conclude that the Z-scheme electron transfers from the CB of SiC to the valence band (VB) of Cu 2 O would be accelerated by the Pt nanoparticles located between Cu 2 O and SiC, due to the excellent conductivity and high work function of Pt. The controlled experiment shows that the Cu 2 O/SiC displays the HCOOH evolution of about 40.5 μmol g −1 h −1 , which is little higher than that of the pristine SiC but much lower than that of Cu 2 O–Pt/SiC samples (Supplementary Fig. 21 ). This means that contribution of the Cu 2 O deposited on SiC surface to the activity is very small, and the high activity is mainly due to the embedding of Pt in the interface between Cu 2 O and SiC. The photocatalytic CO 2 reduction performances of Cu 2 O/SiC/IrO x and Pt–Cu 2 O/SiC/IrO x were also compared with that of Cu 2 O–Pt/SiC/IrO x (Supplementary Fig. 21 ). Much lower activities of Cu 2 O/SiC/IrO x and Pt–Cu 2 O/SiC/IrO x than that of Cu 2 O–Pt/SiC/IrO x indicates likewise that the Pt sandwiched between the interface of Cu 2 O and SiC is more beneficial to the transfer of photogenerated electrons from SiC to Cu 2 O thus enhances CO 2 reduction. Simultaneously, another direct Z-scheme photoelectron transfer occurs at the interface between IrO x and SiC, because SiC has much more positive VB than CB of IrO x . As a result, SiC, Cu 2 O and IrO x in Cu 2 O–Pt/SiC/IrO x all are excited by visible light, the photogenerated electrons from the CB of IrO x (+0.35 V) would transfer towards the VB of SiC (+1.40 V). Synchronously, the photogenerated electrons from the CB of SiC (−1.08 V) would transfer towards Pt nanoparticles, and then towards the VB of Cu 2 O (+0.70 V) where they combine with the photogenerated holes at Cu 2 O. On the whole, the coupled direct Z-scheme processes result in the photogenerated electrons accumulating in the CB of Cu 2 O (−1.28 V) where the adsorbed CO 2 is reduced into HCOOH [ E (CO 2 /HCOOH) = −0.61 V], while the photogenerated holes on the VB of IrO x (t 2g = +1.85 V) to oxidize Fe 2+ into Fe 3+ [ E (Fe 2+ /Fe 3+ )  = +0.77 V] [64] , [65] . Meanwhile, in the H 2 O oxidation chamber, Pt/WO 3 is excited also by visible irradiation. The photogenerated electrons would transfer from the CB of WO 3 (+0.74 V) towards Pt and then reduce Fe 3+ into Fe 2+ [ E (Fe 2+ /Fe 3+ ) = +0.77 V], while the photogenerated holes of WO 3 (+2.06 V) would oxidize H 2 O to O 2 ( E = +1.23 V). As shown in Fig. 9b , the overall photocatalytic system follows indirect Z-scheme mechanism similar to the natural photosynthesis, i.e. the photocatalytic CO 2 reduction half-reaction and the photocatalytic H 2 O oxidation half-reaction take place at two separated reactors by the relaying role of Fe 3+ /Fe 2+ redox couple. To prove that the total reaction is a combination of the spatially separated reduction and oxidation, two controlled experiments were done. When the water solution containing photocatalyst Pt/WO 3 and Fe 3+ is illuminated with visible light, O 2 is generated also as a main product (Supplementary Fig. 22a ), validating the oxidation half-reaction in the left side of Fig. 9b . When the solution containing H 2 O, Cu 2 O–Pt/SiC/IrO x , Fe 2+ and CO 2 is illuminated with visible light, HCOOH is detected also as main product (Supplementary Fig. 22b ), validating the reduction half-reaction in the right side of Fig. 9b . Therefore, Fe 3+ /Fe 2+ redox couple makes the reduction of CO 2 to HCOOH on Cu 2 O–Pt/SiC/IrO x and the oxidation of H 2 O to O 2 on Pt/WO 3 integrated into the one system like the natural photosynthetic systems. It must be mentioned that the usage mode of Fe 3+ and Fe 2+ has little impact on the reaction efficiency. When the Fe 2+ /Fe 3+ mixed solution was used in both cells of the separated reaction system, HCOOH was produced steadily with the reaction time (Supplementary Fig. 23 ), and its generation rate is 629.8 μmol g −1 h −1 . When Fe 2+ and Fe 3+ were separately loaded in the CO 2 -reduction compartment and the H 2 O-oxidation compartment, the initial generation rate of HCOOH is 896.6 μmol g −1 h −1 . Obviously, the separate addition of Fe 2+ solution and Fe 3+ solution in both compartments is more efficient than the loading of Fe 2+ /Fe 3+ mixed solution in both compartments for the photocatalytic reaction in the separated reaction system. But the separated use mode of Fe 2+ and Fe 3+ can only improve initiate photoreaction efficiency. When the redox reaction reaches dynamic steady state, the concentrations of Fe 2+ and Fe 3+ also reach a constant gradient in both sides to maintain counter diffusion. Fe 2+ and Fe 3+ are not evenly dispersed in either cell according to previous study due to osmosis of Fe ions through Nafion membrane [66] . Even though the concentration of Fe 2+ and Fe 3+ is equal in the reaction compartments, the H 2 O oxidation and CO 2 reduction can proceed over the photocatalysts due to the different adsorption property of Fe 2+ /Fe 3+ on photocatalyst surface. For example, Fe 3+ is more favourable to adsorb on WO 3 surface than Fe 2+ (ref. [67] ). Materials SiO 2 and H 2 PtCl 6 ·6H 2 O were acquired from Aladdin, and the Na 3 IrCl 6 was supplied from Alfa Aesar. Other reagents used in this work, including glucose, methanol, WO 3 , NaOH, CuSO 4 ·5H 2 O and NaIO 3 were of analytical reagent grade and obtained from Sinopharm Chemical Reagent Co., Ltd. All of the above chemicals were used without further purification. Preparation of Pt/SiC photocatalyst The SiC nanoparticles were prepared by the carbothermic reduction method. Powders of SiO 2 and glucose were mixed in the molar ratio of Si:C = 1:6 and pulverized in a mortar to well disperse the mixed powders. The well-mixed powder was calcined under Ar atmosphere at 1450 °C for 5 h at a rate of 2 °C min −1 in a tubular furnace. The calcined powder was then cooled to room temperature and further purified to remove unreacted raw materials based on our previous report [26] . Briefly, the sample was calcined under O 2 atmosphere at 873 K for 5 h and steeped with 10 wt% sodium hydroxide solution in order to remove free carbon and unreacted SiO 2 . Platinum (Pt) was loaded on SiC by the photodeposition method as described in the following steps. The H 2 PtCl 6 solution with a concentration of 1 mmol L −1 was mixed with SiC powder in a quartz cell. In the process of stirring, 2 mL of methanol was added into the mixture. After evacuation, the suspension was irradiated with a 125 W Hg lamp to load Pt nanoparticles onto the SiC. After a certain irradiation time, the obtained sample was washed thoroughly with deionized water and dried in vacuum for 1 h. The irradiation time was changed from 0.5 to 2 h to tune the content of Pt in sample, which was denoted as Pt− x h/SiC ( x = 0.5, 1, 1.5, 2, representing the irradiation time). Preparation of Cu 2 O–Pt/SiC and Pt/SiC/IrO x photocatalysts Cu 2 O–Pt/SiC and Pt/SiC/IrO x photocatalysts were also prepared by the similar procedure by using Pt/SiC (Pt-1h/SiC) instead of pure SiC. In the preparation of Cu 2 O–Pt/SiC, CuSO 4 ·5H 2 O aqueous solution in the concentration of 0.6 mmol L −1 and 2 mL of methanol were introduced to the quartz cell together with Pt/SiC. The content of Cu species in the final sample was controlled by changing the irradiation time from 1 to 10 h, the resulting sample was denoted as Cu 2 O–Pt− y h/SiC ( y = 1, 3, 5, 8, 10). For the synthesis of Pt/SiC/IrO x , Na 3 IrCl 6 and NaIO 3 aqueous solution with the respective concentration of 0.6 and 0.01 mol L −1 were added into the reactor to mix with Pt/SiC. The content of Ir species in the final sample was adjusted also by the irradiation time from 1 to 10 h, the resulting sample was denoted as Pt/SiC/IrO x − y h ( y = 1, 3, 5, 8, 10). After IrO x photodeposition, the samples were washed by deionized water and ethanol for several times to remove residual iodine species. The final sample was obtained after drying in vacuum for 1 h. In order to detect the residual iodine ions, the samples were immersed in the AgNO 3 solution. However, we did not find any precipitates AgIO 3 or AgI in solution, indicating iodine ion can be completely washed away in the synthesis process. Preparation of Cu 2 O–Pt/SiC/IrO x photocatalysts Pt/SiC was added to the aqueous solution with CuSO 4 ·5H 2 O (0.6 mmol L −1 ) and Na 3 IrCl 6 (0.6 mmol L −1 ) followed by evacuation and irradiating with a 125 W Hg lamp. The content of Cu and Ir species in the final sample was controlled by the irradiation time from 3 to 15 h. The obtained sample was washed thoroughly with deionized water and dried in vacuum for 1 h, which was denoted as Cu 2 O–Pt- z h/SiC/IrO x ( z = 3, 5, 8, 10,12, 15). Preparation of Pt/WO 3 photocatalyst Pt/WO 3 photocatalyst was also prepared by the photoreduction method similar to that in preparation of Pt/SiC photocatalyst with the irradiation time of 0.5 h. Characterization of photocatalysts XRD patterns were recorded with Ni filtered Cu Kα radiation at 40 kV and 40 mA on a Bruker D8 Advance X-ray diffractometer. Morphology of sample was characterized by a field emission scanning electron microscopy (JSM-6700F) and TEM. TEM images were obtained at an accelerating voltage of 200 kV using a JEOL model JEM 2010 EX instrument. UV–Vis diffuse reflectance (UV–Vis DRS) spectra were obtained on a UV–Vis spectrophotometer (Cary 500) with a self-supporting sample cell, and the pure BaSO 4 was used as a reflectance standard. Brunauer–Emmett–Teller (BET) surface area was measured with an ASAP2020M apparatus (Micromeritics Instrument Corp., USA). Nitrogen adsorption and desorption isotherms were measured at 77 K. Contents of Pt, Cu and Ir in the samples were measured using an inductively coupled plasma optical emission spectrometer (Ultima 2, HORIBA Jobin Yvon Co., France). HS-LEIS measurements were carried out on an IonTOF Qtac100 low-energy ion scattering analyser. 4 He + ions with a kinetic energy of 3 keV were applied at a low ion flux equal to 1325 pA cm −2 , which was necessary to avoid the sputtering of surfaces. 20 Ne + ions with a kinetic energy of 5 keV were applied at a low ion flux equal to 445 pA cm −2 . The scattering angle was 145°. XPS measurements were performed on a Quantum 2000 Scanning ESCA Microprobe (Physical Electronics) using Al Kα radiation (1846.6 eV) as the X-ray source. 13 C NMR spectra were recorded on AVANCE III 400 MHz spectrometer using TMS as the internal standard. 13 CO 2 and H 2 18 O were employed as the reactants in the isotope labelling comparison reaction instead of CO 2 and H 2 O, respectively. After irradiation, the reaction solution was characterized with 13 C NMR directly. FT-IR experiments were carried out on a Nicolet 670 FT-IR spectrometer at a resolution of 4 cm −1 and 64 scans. FT-IR experiments were performed in a home-made IR cell in conjunction with a vacuum system. The catalyst powders were first pressed into a self-supporting disk (18 mm diameter, 20 mg), and then the disk was placed in the sample cell, which allowed the disk to move vertically along the cell tube. Prior to the FT-IR measurements, the disk was treated under a dynamic vacuum (10 −4 Torr) at 473 K for 2 h. After cooling the disk to room temperature, CO 2 was introduced into the cell via the septum with a syringe. Photoluminescence excitation spectra was recorded on a FL/FS920 spectrofluorimeter (Edinburgh Instruments) fluorescence spectrometer at room temperature; the excitation wavelength is 375 nm. CO 2 photoreduction apparatus and reactions The spatially separated Z-scheme system includes a CO 2 -reduction chamber and an O 2 -generation chamber that are divided by a Nafion membrane (The circular Nafion membrane was Fe-ion exchanged before used in the reactor.) (Supplementary Fig. 6 ). The cubage of each reaction chamber is 300 mL. The aqueous solution containing 50 mg photocatalyst (SiC, Pt/SiC, Cu 2 O–Pt/SiC, Pt/SiC/IrO x or Cu 2 O–Pt/SiC/IrO x ) and 2 mM FeCl 2 and another aqueous solution containing 100 mg Pt/WO 3 and 2 mM FeCl 3 were added to the two reaction chambers, respectively. The pH of solutions was adjusted to 2.3 by adding hydrochloric acid to prevent hydrolysis of the iron ions. Prior to irradiation, ultra-pure Ar (99.9995 v%) gas was bubbled through the solution to purge any dissolved air in the O 2 -generation compartment and filled to atmospheric pressure, while ultra-pure CO 2 gas was bubbled through the solution in the CO 2 -reduction chamber and filled to atmospheric pressure. During the photoreaction, the solution in each chamber was stirred and irradiated with a 300 W xenon (Xe) lamp. The lamp with an optical filter ( λ ≥ 420 nm) was vertically placed at equal distance from each chamber, which makes both solutions to receive the same amount of visible light intensity. The solution in the CO 2 -reduction chamber was sampled every 2 h and analysed by ion chromatography (IC, Thermofisher ICS 1100) after filtering catalyst. The gaseous products in O 2 evolution chamber were sampled every 2 h by an off-line sampling syringe (0.5 mL) and then analysed by the gas chromatography (GC, Agilent 7890B, TCD detector) using ultra-pure Ar as the carrier gas. Photoelectrochemical measurements Photoelectrochemical measurements were carried out with a BAS Epsilon workstation using a standard three-electrode electrochemical cell with a working electrode, a platinum foil as the counter electrode, and a saturated Ag/AgCl electrode as the reference. A sodium sulfate solution (0.2 M) was used as the electrolyte, and a 300 W Xe lamp ( λ = 320–780 nm) as the light source. The working electrode was prepared by FTO glass pieces, which was cleaned by sonication in cleanout fluid, acetone and ethanol in sequence prior to use. The photocatalyst was dispersed in ethanol under sonication to form a suspension. A photocatalyst film was fabricated by spreading the suspension onto the conductive surface of the FTO glass.